Redox activity of surface oxygen anions in oxygen-deficient perovskite oxides during electrochemical reactions Surface redox-active centres in transition-metal oxides play a key role in determining the efficacy of electrocatalysts. The extreme sensitivity of surface redox states to temperatures, to gas pressures and to electrochemical reaction conditions renders them difficult to investigate by conventional surface-science techniques. Here we report the direct observation of surface redox processes by surface-sensitive, operando X-ray absorption spectroscopy using thin-film iron and cobalt perovskite oxides as model electrodes for elevated-temperature oxygen incorporation and evolution reactions. In contrast to the conventional view that the transition metal cations are the dominant redox-active centres, we find that the oxygen anions near the surface are a significant redox partner to molecular oxygen due to the strong hybridization between oxygen 2 p and transition metal 3 d electronic states. We propose that a narrow electronic state of significant oxygen 2 p character near the Fermi level exchanges electrons with the oxygen adsorbates. This result highlights the importance of surface anion-redox chemistry in oxygen-deficient transition-metal oxides. Electrochemical reactions involving oxygen gas molecules, such as those occurring at the air electrodes of fuel cells, electrolysers and metal-air batteries, are ubiquitous in energy conversion and storage technologies. A particularly important class of oxygen electrochemical reactions is one that simultaneously reduces oxygen molecules to and incorporates them as solid-state oxygen ions and vice versa [1] . The global oxygen incorporation reaction into lattice vacancies in a crystalline solid [2] is written in Kroger–Vink notation as: where V O denotes oxygen vacancies. This reaction involves a concerted incorporation of molecular oxygen into the solid, and electron transfer ( Fig. 1a ). The electron-transfer step has been proposed to be rate determining [3] , [4] , [5] . Such a two-way traffic of ions and electrons is significantly more complex and less understood than electrochemical reactions occurring at the interface between a liquid electrolyte and a metal or semiconductor electrode, where electrons are the only species transferred between the redox species in solution and the solid ( Fig. 1b ) [1] , [6] . In bulk materials, the oxygen incorporation reaction generally takes place at temperatures >500 °C because of the high activation barrier for oxygen-ion hopping in the solid state. In nanostructured materials, however, oxygen incorporation at room temperature has been demonstrated [7] , [8] . Regardless of the length scales of materials, electrochemical reactions on oxygen-deficient oxides likely involve the formation and annihilation of surface oxygen vacancies under most environmental conditions [9] . 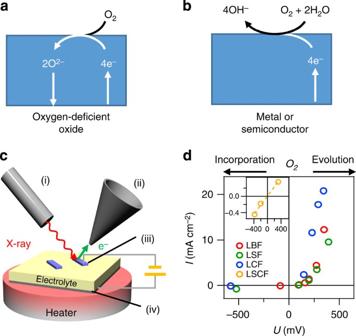Figure 1: Schematic of electrochemical reactions and experimental configuration. (a,b) Comparison of the two-way traffic of ions and electrons in an oxygen-deficient oxide electrode to the electron transfer in a metal or semiconductor electrode (shown here for an alkaline electrolyte). (c) The experimental set-up consists mainly of the X-ray source (i), the differentially pumped electron analyzer (ii), the thin-film perovskite working electrode (iii) and the counter electrode (iv) separated by yttria-stabilized zirconia solid electrolyte. (d) Current–voltage characteristics. (La,AE)FeO3electrodes show a current-limited behaviour under cathodic polarizations due to bulk carrier depletion. The temperature was 550 °C for the ferrite series and 490 °C for LSCF. The oxygen partial pressure for all measurements was 1 Torr. Figure 1: Schematic of electrochemical reactions and experimental configuration. ( a , b ) Comparison of the two-way traffic of ions and electrons in an oxygen-deficient oxide electrode to the electron transfer in a metal or semiconductor electrode (shown here for an alkaline electrolyte). ( c ) The experimental set-up consists mainly of the X-ray source (i), the differentially pumped electron analyzer (ii), the thin-film perovskite working electrode (iii) and the counter electrode (iv) separated by yttria-stabilized zirconia solid electrolyte. ( d ) Current–voltage characteristics. (La,AE)FeO 3 electrodes show a current-limited behaviour under cathodic polarizations due to bulk carrier depletion. The temperature was 550 °C for the ferrite series and 490 °C for LSCF. The oxygen partial pressure for all measurements was 1 Torr. Full size image Transition-metal (TM) oxides with the perovskite crystal structure, typically those based on Mn, Fe, Co and Ni, are widely investigated as air electrodes for solid-oxide [4] and aqueous fuel cells and electrolyzers [10] , and are used as model systems to understand oxygen reactions [11] , [12] . Beyond electrochemical applications, these oxides are also employed to catalyze heterogeneous reactions such as methane reforming [13] and selective dehydrogenation of ethane [14] . Chemical intuition arising from the redox behaviour of TM cations suggests that they are the redox partner to molecular oxygen during electrochemical reactions. For example, in defect models describing perovskites, the redox activity is assigned overwhelmingly to a valence change of the TM cations [15] , [16] , [17] . However, ex situ investigation of bulk TM oxides revealed that hybridization of the TM3 d and O2 p orbitals can give rise to bonds with significant covalent character [18] , [19] , [20] , and the degree of covalency influences the catalytic activity [19] . It has also been found that the covalency of the surface atoms is different than in the bulk [21] . These evidences suggest that the classic ionic picture of surface redox electrochemistry may be insufficient. An overwhelming majority of experimental and computational efforts on perovskite electrodes have aimed at connecting bulk properties to the surface oxygen incorporation rates. For example, a relationship between the surface oxygen exchange rate constants and bulk oxygen-ion diffusion coefficient was observed experimentally [4] , [22] . Using density-functional calculations, Lee et al . [23] also identified a correlation between the surface exchange rate constant and the bulk oxygen vacancy formation energy as well as the bulk O2 p -band centre. In perovskite oxides for aqueous oxygen reduction and evolution reactions at room temperature, the filling of the bulk e g band (arising from the TM-O 6 octahedral field) and the O2 p centre was proposed to serve as descriptors for the electrocatalytic activity [10] , [24] . While these bulk studies have produced valuable insights, the redox nature of the electrochemically active surface remains elusive. This is largely due to the lack of understanding of electrode surfaces under redox-active conditions. In this work, we probe the surface electronic structure of (La,AE)TMO 3−δ electrodes with Fe and Co as TM cations and Ca, Sr or Ba as the alkaline-Earth (AE) substituents under oxygen incorporation and evolution reaction conditions at elevated temperatures. We directly observe redox-active centres on the surface of perovskite oxides thin-film microelectrodes using ambient pressure X-ray absorption spectroscopy (XAS) [25] in a highly surface-sensitive detection mode. By probing the electronic structure of both surface lattice oxygen and TM ions during reaction 1, we show that oxygen is a significant redox partner to the oxygen adsorbate, where a narrow electronic state of considerable O2 p character on the perovskite surface is populated and depopulated. The importance of anion-redox chemistry in oxygen-deficient metal-oxide electrocatalysts, particularly that arising from the localized electronic states on oxygen, challenges the current paradigm of electrocatalyst design, which has been focused largely on the cation redox chemistry. Electrochemical polarization Highly textured thin-film microelectrodes of La 0.5 Sr 0.5 FeO 3−δ (LSF), La 0.5 Ca 0.5 FeO 3−δ (LCF), La 0.5 Ba 0.5 FeO 3−δ (LBF) and La 0.6 Sr 0.4 Co 0.2 Fe 0.8 O 3−δ (LSCF) (nominal compositions) were deposited by pulsed-laser deposition (PLD) on yttria-stabilized zirconia single crystals, which also serve as the oxygen-ion-conducting solid electrolyte ( Fig. 1c , see Supplementary Methods for fabrication details and additional characterizations). The topmost atomic layers of electrochemical cells were probed operando with partial-electron-yield XAS at 1 Torr O 2 and at 550 °C (LSF, LCF and LBF) and 490 °C (LSCF). The information depth is estimated to be on the order of 1 nm (see Supplementary Methods ). In contrast to high-vacuum experiments, the environmental conditions employed here are beginning to approach those of technologically relevant solid-oxide fuel cells and electrolyzers. At these conditions, the perovskite electrodes exhibit mixed oxygen-ion and electron–hole conductivity [17] . Cathodic (negative) and anodic (positive) biases were applied to the perovskite electrode to drive the oxygen incorporation and evolution reactions, respectively. Figure 1d shows the current–voltage characteristics of the electrochemical cells determined during the XAS measurements.To assess the overpotential of the electrode under applied bias, we carried out X-ray photoelectron spectroscopy alongside the XAS to quantify shifts of various core-level photoelectron peaks (with the electrode Fermi-coupled to the electron analyzer, and a probing depth of ~1 nm, similar to the XAS) [6] , [26] . We observed that all photoelectron peaks shift rigidly with the applied bias, confirming that the electron chemical potential in the electrodes are changing without a substantial change in the lattice energy. Moreover, a nearly one-to-one relationship between the binding energy shift and the Ohmic-corrected overpotential was observed ( Fig. 2 ). This confirms that the majority of the overpotential occurs at the perovskite/oxygen interface. For the LSCF electrode, we employed an in-plane electrochemical cell, and in addition verified that the bias-dependent potential difference between the perovskite electrode and the solid electrolyte (given by the kinetic energy of the Zr 3 d photoelectron peak at a location immediately next to the electrode) matches the Ohmic-corrected overpotential ( Supplementary Fig. 1 ). 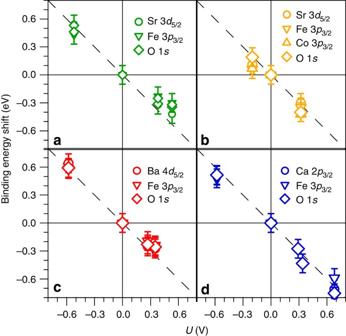Figure 2: Core-level binding energy shifts as a function of ohmic-corrected bias. Shifts are measured by X-ray photoelectron spectroscopy for LSF (a), LSCF (b), LBF (c) and LCF (d). The binding energy shifts are referenced to open-circuit conditions. The dashed lines mark the 1:1 relationship. All core-level peaks shift rigidly, indicating a shift in the Fermi level upon polarization. The error bars on thex-axis represent the uncertainty of the photon energy of 0.1 eV. Given this observation, we take the Ohmic-corrected bias as the electrode overpotential. Figure 2: Core-level binding energy shifts as a function of ohmic-corrected bias. Shifts are measured by X-ray photoelectron spectroscopy for LSF ( a ), LSCF ( b ), LBF ( c ) and LCF ( d ). The binding energy shifts are referenced to open-circuit conditions. The dashed lines mark the 1:1 relationship. All core-level peaks shift rigidly, indicating a shift in the Fermi level upon polarization. The error bars on the x -axis represent the uncertainty of the photon energy of 0.1 eV. Given this observation, we take the Ohmic-corrected bias as the electrode overpotential. 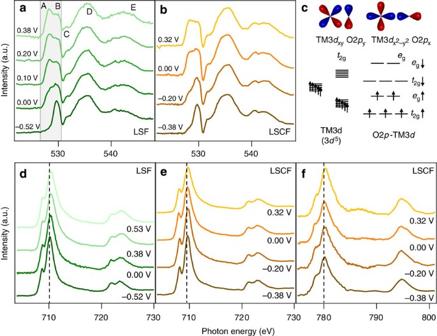Figure 3: Operando oxygen K-edge and TM L-edge X-ray absorption spectra. (a) LSF and (b) LSCF O-K-edge and transition-metal L-edge spectra of (d) LSF and (e,f) LSCF at various overpotentials. (c) Schematic of the orbital arrangement of the TM3d-O2pmanifold in an octahedral field in the high spin state. The O K-edge absorption features are assigned as follows: (A) hybridized TM3d-O2p eg↑, (B)t2g↓, (C) oxygen gas absorption dip, (D) (La,alkaline-Earth)5/4d-O2pand (E) TM4sp-O2pstates. Full size image Oxygen K-edge spectroscopy Figure 3a,b shows the X-ray absorption spectra at the O K-edge under a wide range of overpotentials for LSF and LSCF. Spectra for additional compositions are shown in Supplementary Fig. 2 . The prominent dip at 530.8 eV (labelled ‘C’) is due to X-ray absorption by the oxygen gas molecules, the partial pressure of which is held constant throughout the experiment. We show that this feature does not affect the region of analysis ( Supplementary Fig. 3 ). Figure 3 also shows the Fe L-edge spectra, as well as the Co L-edge spectra for LSCF. TM spectra of additional compositions are shown in Supplementary Fig. 4 . To confirm the reversibility of the electrode surface, we compared the O K-edge and Fe L-edge spectra at the open-circuit condition before and after the measurement ( Supplementary Fig. 5 ). The difference plot shows negligible change upon electrochemical cycling, confirming the reversibility of the electrode surface. Figure 3: Operando oxygen K-edge and TM L-edge X-ray absorption spectra. ( a ) LSF and ( b ) LSCF O-K-edge and transition-metal L-edge spectra of ( d ) LSF and ( e , f ) LSCF at various overpotentials. ( c ) Schematic of the orbital arrangement of the TM3 d -O2 p manifold in an octahedral field in the high spin state. The O K-edge absorption features are assigned as follows: (A) hybridized TM3 d -O2 p e g ↑, (B) t 2g ↓, (C) oxygen gas absorption dip, (D) (La,alkaline-Earth)5/4 d -O2 p and (E) TM4 sp -O2 p states. Full size image Both Fe and Fe-Co perovskite electrodes show very similar behaviour: the O K-edge spectra, particularly the pre-edge regions between ~525 and 530 eV (highlighted in Fig. 3a ), exhibit a clear and systematic dependence on overpotential. For the TM absorption spectra, on the other hand, spectral shapes and the positions of the white line (photon energy at which maximum absorption occurs) appear largely invariant with overpotential. First, we discuss the features in the O K-edge absorption spectra, labelled A–E in Fig. 3a . Only spectral features ‘A’ and ‘B’ exhibit a clear dependence on the applied overpotential, which are shown enlarged in Fig. 4a,b . In theory, these features could arise from physisorbed oxygen, as well as lattice oxygen associated with possible precipitated oxide phases on the surface (typically AE oxide islands [27] ). As we discuss in the Supplementary Methods , these candidate species show spectroscopic signatures at significantly higher photon energies than that of overpotential-dependent features ‘A’ and ‘B’. Thus, we assign these features to intrinsic electronic states within the perovskite phase based on previous reports of bulk LSF [28] , where Fe is in the high spin configuration: the features ‘A’ and ‘B’ are assigned to unoccupied states of Fe/Co3 d -O2 p mixed character generated by the hybridization of Fe/Co3 d and O2 p in the octahedral crystal field. This forms e g and t 2g molecular orbitals, which represent σ and π TM–O bonds, respectively (see Fig. 3c ). Specifically, feature ‘A’ corresponds to the e g ↑ states and feature ‘B’ to the t 2g ↓ states. The energetically higher e g ↓ states are convoluted with the gas absorption peak ‘C’ and thus will not be discussed further. A contribution of the e g ↓ state to feature B due to close proximity in absorption energy cannot be excluded completely, but does not affect our analysis, as we show later. We also assign ‘D’ to electronic states of La/AE5/4 d -O2 p character, and the broad feature ‘E’ to Fe/Co4 sp -O2 p states. We note that the addition of Co to the system does not affect the shape or position of the features observed in the O K-edge ( Fig. 4 ), making Co–O and Fe–O states indistinguishable spectroscopically. 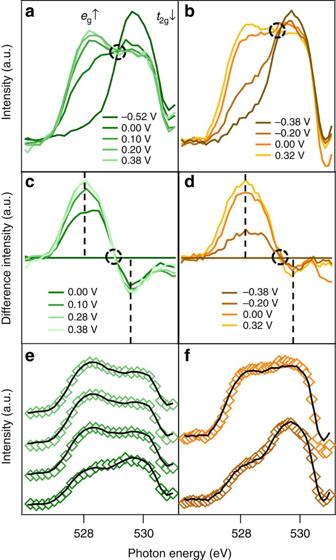Figure 4: Analysis of O K-edge absorption spectra. Superimposed O K-edge absorption spectra of (a) LSF and (b) LSCF electrodes at various overpotentials. The isosbestic points are circled. Difference spectra (with respect to the spectra measured under the most cathodic overpotential) for (c) LSF and (d) LSCF. The dashed lines mark the average peak position and indicate the peaks corresponding toeg↑ andt2g↓ states do not vary in absorption energy with overpotential. The spectra can be described as a linear combination of two end-member spectra (ones corresponding to the most anodic and cathodic overpotentials): (e) LSF and (f) LSCF. Open markers indicate data and solid lines indicate linear combination fits. SeeSupplementary Figs 6–8for analysis on additional electrode compositions. Figure 4: Analysis of O K-edge absorption spectra. Superimposed O K-edge absorption spectra of ( a ) LSF and ( b ) LSCF electrodes at various overpotentials. The isosbestic points are circled. Difference spectra (with respect to the spectra measured under the most cathodic overpotential) for ( c ) LSF and ( d ) LSCF. The dashed lines mark the average peak position and indicate the peaks corresponding to e g ↑ and t 2g ↓ states do not vary in absorption energy with overpotential. The spectra can be described as a linear combination of two end-member spectra (ones corresponding to the most anodic and cathodic overpotentials): ( e ) LSF and ( f ) LSCF. Open markers indicate data and solid lines indicate linear combination fits. See Supplementary Figs 6–8 for analysis on additional electrode compositions. Full size image Because alkaline-metal cations are known to rearrange at elevated temperatures [27] , [29] , [30] , we investigated the effect of such rearrangements on the surface electronic structure. Specifically, the accumulation and depletion of AE ions can influence the electron–hole concentration as required by electroneutrality. In turn, variation in the hole concentration can modulate the pre-edge features A and B in the O K-edge XAS. We performed an upper-bound analysis, whereby we assume that all Sr enrichment and La/Sr vacancies (determined by XPS measured alongside with the XAS) are charge compensated by electron–holes (see Supplementary Methods and Supplementary Figs 9–13 ). The analysis shows that Sr enrichment and La/Sr vacancies only accounts for a minority fraction of the electron–holes generated. Therefore, we propose that electron-holes generated on the surface are charge compensated primarily by the annihilation of oxygen vacancies (i.e., via reaction 1). The lowest energy absorption feature corresponding to unoccupied e g ↑ state increases in intensity with anodic polarizations (oxygen-evolution conditions). This behaviour is consistent with the depopulation of electronic states near the Fermi level (and vice versa under cathodic polarizations). Such a change in the electron concentration takes place side by side with the annihilation of oxygen vacancies (see reaction 1), and corresponds to an oxidation of the perovskite and a lowering of the Fermi level. Even in the absence of quantitative analysis, the clear and systematic dependence of the e g ↑ peak intensity on overpotential (attributed to the O2 p states hybridized with the TM3 d states) strongly suggests that the oxygen is redox active in Fe and Fe-Co perovskites during oxygen incorporation and evolution. Moreover, the surface of the perovskite remains redox active even under relatively large overpotentials, and does not exhibit Fermi level pinning as observed in certain semiconductor electrodes in aqueous systems [31] . As the perovskite electrodes become more oxidized under oxygen-evolution reaction conditions (corresponding to a lowering of the Fermi level, see Fig. 2 ), the O K-edge absorption threshold does not shift. When depicted as difference spectra in Fig. 4c,d , it is clear that the absorption peaks vary in intensity but not in the absorption energy. This observation contrasts with previous reports of LaCoO 3−δ , where the O K-edge absorption threshold shifts towards lower photon energy gradually with Sr doping when reaching the metallic regime at high Sr concentration [32] . Such a shift also has been observed for homovalent TM substitution across the semiconductor to metal transition [33] , and likewise for LSF by Abbate et al . [28] , though the peak shifts are somewhat small. The absorption threshold corresponds to the energy of the lowest unoccupied electronic states. When these states are close to the Fermi level (in the order of the thermal voltage) and are large in bandwidth, the energy of the lowest unoccupied electrons shifts continuously with Fermi level. When these states are small in bandwidth, on the other hand, the states are filled or unfilled without a significant change in the energy of the lowest unoccupied electronic states. Our observation suggests that the latter is the case in the perovskite electrodes investigated: a narrow electronic state is populated and depopulated near the Fermi level during oxygen reduction and evolution reactions. This is consistent with the small-polaron conduction mechanism via localized electronic charge carriers in AE-substituted LaFeO 3−δ at elevated temperatures [17] , [34] , [35] . The proposed electronic structure, depicted schematically in Fig. 5e , differs from previous observation in bulk Fe-SrTiO 3 , where the redox-active Fe states overlap with the top of the valence band, and a broad valence band is filled and emptied [36] . 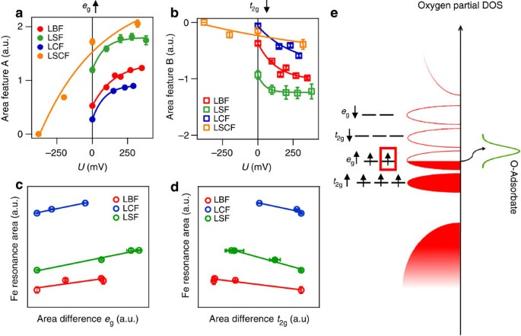Figure 5: Quantitative analysis of absorption spectra and proposed oxygen band structure. Area under the curve for (a)eg↑ and (b)t2g↓ peaks for the difference spectra presented inFig. 4c,d, shown for Ba, Sr and Ca-substituted LaFeO3and LSCF electrodes. Lines are guide to the eye. (c,d): correlation of Fe L-edge resonance area to theeg↑ andt2g↓ difference areas shown in (a,b,e) Schematic band structure of the oxide, showing only the oxygen partial density of states (DOS). The bandwidths are shown schematically. A contribution of theeg↑ andeg↓ state to feature B cannot be excluded completely. Error bars are the s.e. as determined from the s.d. of the individual data points of the spectra. Figure 5: Quantitative analysis of absorption spectra and proposed oxygen band structure. Area under the curve for ( a ) e g ↑ and ( b ) t 2g ↓ peaks for the difference spectra presented in Fig. 4c,d , shown for Ba, Sr and Ca-substituted LaFeO 3 and LSCF electrodes. Lines are guide to the eye. ( c , d ): correlation of Fe L-edge resonance area to the e g ↑ and t 2g ↓ difference areas shown in ( a , b , e ) Schematic band structure of the oxide, showing only the oxygen partial density of states (DOS). The bandwidths are shown schematically. A contribution of the e g ↑ and e g ↓ state to feature B cannot be excluded completely. Error bars are the s.e. as determined from the s.d. of the individual data points of the spectra. Full size image To further support the conclusion that the electronic states accessed during oxygen incorporation and evolution are narrow in bandwidth, we take a closer look at the superimposed O K-edge spectra ( Fig. 4a,b ). An isosbestic point (a common intersection point for all spectra) is clearly evident for all compositions investigated. Moreover, the isosbestic point manifests itself as a common zero-crossing point in the difference spectra shown in Fig. 4c,d . The observation of this isosbestic point motivated us to fit each spectrum as a linear combination of two end-member spectra, one for the most oxidized and one for the most reduced state accessed in our experiments. Indeed, O K-edge spectra for all samples at every applied overpotential can be described very well using this linear combination analysis ( Fig. 4e,f ). This indicates that an observed spectrum could be the sum of two and only two spectra [37] , representing the mostly filled and empty oxygen redox state. Interestingly, the O K-edge absorption spectroscopy indicates that the degree of surface oxidation and reduction is similar between LSF and LSCF ( Fig. 4 , and further quantified in Fig. 5a ), both at open-circuit and under electrochemical polarization. This observation is surprising because the oxygen vacancy formation energy in bulk LSCF is known to be significantly less than in bulk LSF [38] . Our results confirm that the energetics of surface reduction (and oxidation) in perovskite can differ substantially from those of the bulk, consistent with predictions that oxygen vacancy forms more easily on the surface of perovskites than in the bulk [39] . This observation highlights the importance of surface-sensitive, operando measurements of the electronic structure. TM L-edge spectroscopy Turning to the Fe L-edge absorption spectra in the (La,AE)FeO 3−δ electrodes, the variation with overpotential is less pronounced than the O K-edge ( Supplementary Fig. 14 ). Specifically, the energy of maximum absorption (white line) shifts by no more than 0.16 eV (with the reproducibility of the photon energy ~±0.1 eV), and the intensity ratio of the two L 3 features is essentially independent of overpotential. There is, however, a subtle decrease in the overall intensity of the iron white lines with overpotential, accompanied by a broadening of the high-energy tail of the L 3 edge. In the LSCF electrode which contains both Fe and Co, on the other hand, the variation in the TM absorption spectra is greater than the (La,AE)FeO 3−δ electrodes. Specifically, the variation of the intensity ratio of the two L 3 features suggest a more significant change in the Co and Fe valence compared with Fe in (La,AE)FeO 3−δ . Overall, the constant white line position in the Fe L-edge spectra with overpotential is similar to spectroscopy of prior bulk LSF studies, where oxygen vacancies are generated by aliovalent substitution [28] or by chemical oxidation/reduction [20] . Similar observation was also made on Fe-doped BaZrO 3 (ref. 40 ). It is generally accepted that the lack of major change in the TM absorption spectra arises from the strong oxygen character of the TM–O bond, consistent with our interpretation that oxygen is redox active. From models developed to describe correlated electron systems, our observations here can be explained by the fact that the charge-transfer energy is lower than the Mott-Hubbard energy [41] , rendering the electrodes to be low charge-transfer energy oxides [42] , [43] . As a result, the electron–holes are located on states of predominantly O2 p character, leading to a transition from a 3 d 5 to a 3 d 5 L configuration where L denotes a ligand hole. Moreover, our results indicate that the Fe 3+ /Fe 4+ state (changing from d 5 to d 4 ) is too far from the Fermi level to be accessed even when electrochemically oxidizing the material with large anodic overpotentials. Our observation is consistent with recent work on BaFeO 3 (ref. 44 ) and Fe-doped BaZrO 3 (ref. 40 ), where an Fe 4+ oxidation state could not be obtained under highly oxidizing conditions. Effect of covalency Finally, we quantified the evolution of the e g ↑ and t 2g ↓ absorption features in the O K-edge spectra by numerically integrating the area of the difference plots for these states. The general trend is very similar in both the Fe and mixed Fe-Co perovskites: the e g ↑ absorption feature grows with anodic polarizations ( Fig. 5a ), whereas the t 2g ↓ absorption feature declines ( Fig. 5b ). Because both absorption features can be readily described by the same linear combination analysis, they must arise from a highly coupled phenomenon. However, this observation cannot be explained by simple population and depopulation of electronic states because the relatively energetic t 2g ↓ state cannot be readily accessed during surface redox processes. We propose that while the variation in the e g ↑ absorption features principally results from population and depopulation of electronic states near the Fermi level, the variation in the t 2g ↓ absorption feature corresponds to a change in the degree of covalency. This concerted effect can be explained with the O2 p /TM3 d orbital arising from the ligand being the active redox state; the population of this state during the reaction will have an effect on covalency. To explore this hypothesis, we analyze the total integrated areas of the oxygen and iron spectra (that is, the spectroscopic resonances), which are correlated with the degree of covalency [45] ( Supplementary Fig. 15 ). We note, however, changes in the oxidation state may also impact the shape and resonance of the spectra. For the A-site-substituted LaFeO 3−δ electrodes, the Fe spectroscopic resonances show a trend of greater area (decreased covalency of the Fe–O bond) with increasing anodic overpotential. This is consistent with the decline of the t 2g ↓ spectral feature. Indeed, the Fe resonances are linearly correlated to the differential t 2g ↓ population and likewise for the e g ↑ population ( Fig. 5c,d ). Moreover, our observation is in line with a study where the covalency changes as a function of e g ↑ electron count induced by B-site substitution [19] . With a decline in the Fe resonance, we would also expect an increase in the total integrated area of the oxygen spectra, which indicates the growing oxygen character of the TM–O bond. However, this was not observed, and is explained by the fact that the integrated O K-edge spectral area is affected not only by the covalency, but also by the population and depopulation of states during oxygen incorporation and evolution. While not definitive, this observation lends support to our hypothesis that the (de)populating of the e g ↑ state is a process coupled with the change in covalency. The variation in covalency in the (La,AE)FeO 3−δ electrodes can also explain the broadening of the high-energy tail of the L 3 edge and a rise in intensity for the second feature of the L 2 peaks under cathodic overpotentials, as shown in calculated line shapes [46] . We note that the above analysis does not extend easily to LSCF, where the TM–O bond involves three species (Fe, Co and O) which results in a complex electron redistribution. In summary, by carrying out surface-sensitive XAS on perovskite-oxide thin-film electrodes during oxygen incorporation and evolution, we determined the redox states of surface TM and oxygen ions under conditions relevant to solid-oxide fuel cells and electrolyzers. We found that the surface lattice oxygen anion is a key redox partner to molecular oxygen. Thus, during oxygen incorporation, surface lattice oxygen is oxidized while the oxygen adsorbate is reduced. Specifically, we observed that the highest unoccupied electronic state is a narrow state of significant O2 p character arising from covalency, which exchanges electrons with the oxygen adsorbate species. As has been shown recently in lithium-ion battery electrodes, bulk anion-redox chemistry is becoming increasingly important [47] , [48] , [49] . Our direct operando observation here confirms that the crucial role of anion-redox chemistry extends to the surface of oxygen-deficient oxides during electrochemical reactions. The fact that the covalent part of the TM–O bond plays an important role shows that an isolated treatment of the redox levels of the cations is insufficient. Rather, the TM-O 6 octahedron as a whole should be considered as the redox-active building block. This opens up novel substitution strategies based on modulating anion-redox chemistry and the anion-TM interaction as avenues to design new electrochemically active materials. Sample preparation Perovskite-oxide thin films were deposited via PLD on 0.5 mm-thick, (001)-oriented, single-side-polished 8 mol% Y 2 O 3 -doped ZrO 2 (YSZ) single crystals (MTI Corp). A 10 mol% Sm 2 O 3 -doped CeO 2 (SDC) buffer layer was also deposited to suppress cation inter-diffusion between YSZ and the perovskite thin film. Two sets of samples were prepared for each material composition: (a) 8.0 × 8.0 mm films deposited on the polished side of the substrate for ex situ characterizations, and (b) complete electrochemical cells with a 0.5 × 2.0 mm 2 perovskite working electrode for the operando X-ray spectroscopy experiments. For the (La,AE)FeO 3−δ electrodes, a cross-plane electrochemical cell was employed: the working electrode was deposited on the polished side of YSZ, and the counter electrode (200-nm-thick Ba 0.5 Sr 0.5 Co 0.8 Fe 0.2 O 3−δ ) was deposited via PLD on the rough side of YSZ, also with a SDC buffer layer. For LSCF, an in-plane cell geometry was employed: both working and counter electrodes (also LSCF) were deposited on the polished side of YSZ. The counter electrode has an area of ~8.0 × 4.0 mm 2 and is separated from the working electrode by 3 mm. The in-plane geometry enabled determination of the overpotential via rigid shifts of the photoelectron peaks as shown in Supplementary Fig. 1 . PLD targets were fabricated via a solid-state reaction route. Appropriate amounts of La 2 O 3 (99.999% purity, Sigma-Aldrich), BaCO 3 (99.999% purity, Sigma-Aldrich)/SrCO 3 (99.994% purity, Alfa Aesar)/CaCO 3 (99.997% purity, Alfa Aesar) and Fe 2 O 3 (99.998% purity, Alfa Aesar)/CoO (99.998% purity, Alfa Aesar) were ground together. The well-mixed powder was then compacted uniaxially at 130 MPa for 10 min into discs 25.4 mm in diameter. The green bodies were subsequently sintered under 21% O 2 balanced with Ar: the furnace was ramped at a rate of 2 °C min −1 to 800 °C, held for 2 h, further ramped at 2 °C min −1 to 1,300 °C (LSF and LCF), 1,200 °C (LBF) or 1,100 °C (LSCF) and held for 10 h. The samples were cooled down at 5 °C min −1 to room temperature. The preparation of the SDC target was described elsewhere [50] . A KrF excimer laser (Lambda Physics LPX200, 248 nm) was employed to deposit the thin films. The (La,AE)FeO 3−δ microelectrodes, the buffer layers and the counter electrodes were deposited at a laser fluency of~1 J cm −2 , a repetition rate of 10 Hz and a substrate-to-target distance of 60 mm. The LSCF electrodes were deposited at 1 J cm 2 and 5 Hz repetition rate at a substrate-to-target distance of 80 mm. The heater temperature for all depositions was set to 800 °C and the deposition atmosphere was 5 mTorr of O 2 . After deposition, the films were cooled down in the same atmosphere at a rate of 5 °C min −1 . Sample characterization X-ray diffraction patterns of the as-deposited thin films ( Supplementary Fig. 16 ) were measured in between 2 θ =20° and 80° (Panalytical Xpert PRO, Cu Kα). The films were confirmed to have the cubic perovskite structure. The out-of-plane θ -2 θ scans show only the (00L) family of peaks, whereas the in-plane φ scans show that the perovskite oxides are rotated 45° crystallographically with respect to the SDC buffer layer and the YSZ substrate. XPS reveals no significant contribution from contaminants such as SiO x , SO x or CO x ( Supplementary Fig. 17 ). Total film thickness (perovskite and SDC buffer layer, Supplementary Table 1 ) was measured by profilometry (Dektak 150, Veeco). The stoichiometry was determined by inductively coupled plasma mass spectrometry (Thermo Scientific XSeries 2) or optical emission spectroscopy (Thermo Scientific ICAP 6300 Duo View). The films were dissolved in aqueous 2% nitric acid. The cation stoichiometries were normalized to either an A- or B-site deficient stoichiometry, as an A- or B-site excess cannot be readily accommodated in the perovskite structure. Operando ambient pressure XAS XAS was carried out at beamline 11.0.2 25 , Advanced Light Source (Lawrence Berkeley National Laboratory) in partial-electron-yield detection mode. The characteristic information depth is estimated to be ~1 nm as elaborated in the Supplementary Methods . The electrochemical cell was placed on a custom sample holder [51] equipped with a ceramic heater and Pt–Ir electrical probes, which contacted the microelectrode. For the cross-plane electrochemical cell, a wound Pt coil, placed between the heater and the cell, contacted the counter electrode. Electrochemical polarization was carried out using biased impedance spectroscopy (Biologic SP-300 potentiostat). The alternating current perturbation was 20 mV at open-circuit condition and is always <5% of the direct current bias. Oxygen reduction reaction was confirmed by a sustained and constant electrochemical current under cathodic polarisation ( Supplementary Fig. 18 ). Temperature was determined using the YSZ ionic resistance, which was calibrated inside the blackbody environment of a tube furnace. XAS normalization was carried out using the ATHENA software [52] . The background was removed from the spectra by fitting a line to the pre-edge range between 520 and 524 eV for oxygen, and between 703 and 706 eV for iron and 770 and 775 eV for cobalt. The spectra were subsequently normalized by fitting a second-order polynomial to the data in the energy range between 550 and 570 eV for oxygen, between 727 and 735 eV for iron and between 800 and 810 eV for cobalt. How to cite this article: Mueller, D. N. et al . Redox activity of surface oxygen anions in oxygen-deficient perovskite oxides during electrochemical reactions. Nat. Commun. 6:6097 doi: 10.1038/ncomms7097 (2015).